Travelling and splitting of a wave ofhedgehogexpression involved in spider-head segmentation During development segmentation is a process that generates a spatial periodic pattern. Peak splitting of waves of gene expression is a mathematically predicted, simple strategy accounting for this type of process, but it has not been well characterized biologically. Here we show temporally repeated splitting of gene expression into stripes that is associated with head axis growth in the spider Achaearanea embryo. Preceding segmentation, a wave of hedgehog homologue gene expression is observed to travel posteriorly during development stage 6. This stripe, co-expressing an orthodenticle homologue, undergoes two cycles of splitting and shifting accompanied by convergent extension, serving as a generative zone for the head segments. The two orthodenticle and odd-paired homologues are identified as targets of Hedgehog signalling, and evidence suggests that their activities mediate feedback to maintain the head generative zone and to promote stripe splitting in this zone. We propose that the 'stripe-splitting' strategy employs genetic components shared with Drosophila blastoderm subdivision, which are required for participation in an autoregulatory signalling network. Animal segmentation, which generates a spatial, periodic pattern, has been studied using various organisms [1] , [2] , [3] and serves as a simple platform to study the mathematical basis of biological pattern formation [4] , [5] , [6] , [7] . 'Subdivision' and 'oscillation' are two major categories of animal segmentation strategies ( Fig. 1a,b ). The former is represented by segmentation of the blastoderm of the long-germ insect Drosophila , which requires a relatively complex readout of morphogen gradients pre-established in a relatively large field and a hierarchy of gene interactions [8] , [9] . The latter is represented by segmentation of the vertebrate paraxial mesoderm, which requires a time-delayed autorepression system that achieves rhythmic oscillation to generate new, solitary, travelling waves successively [1] , [10] , [11] , [12] , [13] . A similar oscillatory mechanism might be involved in the segmentation that occurs sequentially in the posterior growth zone in embryos of short-germ arthropods, such as spiders [14] . 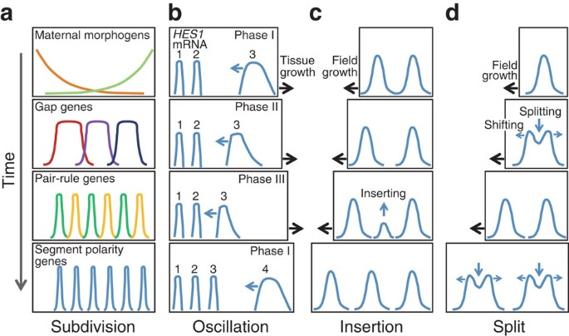Figure 1: Various strategies to generate a spatial periodic pattern. Blue curved lines indicate profiles of authentic or hypothetical segmental gene expression along the axis of the field. Differences are observed in how the new waves originate. (a) 'Subdivision' in segmentation of theDrosophilablastoderm embryo. Hierarchical cascades of maternal morphogens (shown in orange and light green), gap genes (shown in red, purple and dark blue), and pair-rule genes (shown in green and yellow) subdivide the embryo into progressively smaller domains and eventually lead to initiation of the expression of segment polarity genes nearly simultaneously in all of the forming segments8,9. For simplicity, some segments are omitted. (b) 'Oscillation' in segmentation of the mouse paraxial mesoderm. Oscillatory generation of new solitary travelling waves of expression ofHES/hairyfamily genes, such asHES1, develops into a spatial periodic pattern1,10,11,12,13. The number at the peak of each wave indicates the birth order of the waves. (c) 'Insertion' of activator peaks, which has been observed in numerical simulations of reaction–diffusion systems of the activator-inhibitor type on a growing field19,20,21. Note that the new wave arises at a distance from the pre-existing waves. (d) 'Split' of activator peaks, which has been observed in numerical simulations of reaction–diffusion systems of the activator-depleted substrate type on a growing field6,19,22,35. Each cycle of splitting and shifting represents a kind of self-replication. Figure 1: Various strategies to generate a spatial periodic pattern. Blue curved lines indicate profiles of authentic or hypothetical segmental gene expression along the axis of the field. Differences are observed in how the new waves originate. ( a ) 'Subdivision' in segmentation of the Drosophila blastoderm embryo. Hierarchical cascades of maternal morphogens (shown in orange and light green), gap genes (shown in red, purple and dark blue), and pair-rule genes (shown in green and yellow) subdivide the embryo into progressively smaller domains and eventually lead to initiation of the expression of segment polarity genes nearly simultaneously in all of the forming segments [8] , [9] . For simplicity, some segments are omitted. ( b ) 'Oscillation' in segmentation of the mouse paraxial mesoderm. Oscillatory generation of new solitary travelling waves of expression of HES/hairy family genes, such as HES1 , develops into a spatial periodic pattern [1] , [10] , [11] , [12] , [13] . The number at the peak of each wave indicates the birth order of the waves. ( c ) 'Insertion' of activator peaks, which has been observed in numerical simulations of reaction–diffusion systems of the activator-inhibitor type on a growing field [19] , [20] , [21] . Note that the new wave arises at a distance from the pre-existing waves. ( d ) 'Split' of activator peaks, which has been observed in numerical simulations of reaction–diffusion systems of the activator-depleted substrate type on a growing field [6] , [19] , [22] , [35] . Each cycle of splitting and shifting represents a kind of self-replication. Full size image Although mathematical modelling of Drosophila and vertebrate segmentation has been attempted based on experimental observations [15] , [16] , [17] , [18] , further theoretical approaches, particularly numerical analyses of chemical reactions and diffusion, have led to the proposal of different pattern-forming systems that might potentially be applied to animal segmentation. Two-component autocatalytic reaction–diffusion systems may cause successive insertion of new activator peaks between pre-existing activator peaks [19] , [20] , [21] ( Fig. 1c ) and repeated cycles of splitting and shifting of pre-existing activator peaks [6] , [19] , [22] ( Fig. 1d ). Both the insertion and the splitting of activator peaks are promoted by field growth. Although stained embryos, which indicate that a domain of gene expression is resolved into multiple stripes or patches in a relatively short time, have been described [23] , [24] , 'splitting' events in the context of animal segmentation have not been well characterized in cellular and molecular terms. The present work is focused on head segmentation in embryos of the spider Achaearanea tepidariorum . In these embryos, cellularization is complete at or before the 16-nucleus stage [25] , indicating that all of their segmentation processes occur in a cellular environment. The segmented germ band of the embryos is divided into three regions corresponding to the head (cephalon), thorax and opisthosoma. The head bears two pairs of appendages, the chelicerae (Ch) and the pedipalps (Pp), and the thorax has four pairs of appendages, which are the walking legs (L1-4). The A. tepidariorum gene At-hedgehog ( At-hh ) [26] , a homologue of the Drosophila segment polarity hh gene encoding a secreted signalling protein, is expressed on the future anterior side of the embryo [27] . The At-hh expression begins from approximately early stage 3 (ref. 27 ), and later, At-hh serves as an early molecular indicator for head and opisthosomal segmentation [23] , [26] , [27] . Absence of At-hh activity results in severe caudalization [27] . The initial expression of the A. tepidariorum homologue of the Drosophila head gap-like orthodenticle ( otd ) gene, At-otd [28] , requires strong Hh signalling inputs [27] . This At-otd expression is essential for the specification of the entire head region [23] . However, little is known about stripe-forming processes related to spider-head segmentation. In this study, taking advantage of the spider model, we identify 'stripe-splitting' segmentation, which is associated with the convergent extension that elongates the spider-head axis. Based on observations at the cellular and molecular levels, we define a new category of segmentation strategy, split-type segmentation. Functional analyses lead us to propose that split-type spider-head segmentation requires an autoregulatory signalling network in which At-hh , At-otd , and other homologues of Drosophila segmentation genes participate. Travelling of an At-hh stripe To determine where the presumptive head ectoderm is located in the early stage 5-germ disc, we microinjected fluorescent dextran into single blastomeres. Tracking of labelled cell clones revealed that the head ectoderm corresponding to the Ch and Pp segments was derived from germ disc cells that had been located 3–5 cells away from the germ disc rim at early stage 5 ( Fig. 2a,b ). Live observation of a labelled cell clone followed by in situ hybridization revealed that the initial rim cells were internalized during mid-stage 5 to early stage 6, and many but not all of these cells became At-twist ( At-twi )-expressing mesoderm cells [26] , [29] ( Supplementary Fig. S1 and Supplementary Movie 1 ). 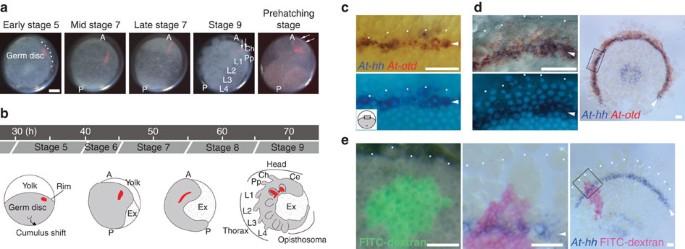Figure 2: Movement of theAt-hhexpression stripe from the rim of the germ disc. (a) Tracking of a small cell clone labelled by microinjection of RITC–dextran (red). The live embryo was photographed at stages indicated. The rim of the germ disc near the clone is dotted (early stage 5). Arrows indicate the developing Ch and Pp segments. (b) Schematic diagram ofAchaearaneadevelopment highlighting the transformation of the germ disc into a segmented germ band. The tracked cell clone shown inais depicted in red. Approximate time after egg laying is shown. (c) Expression ofAt-hh(purple) andAt-otd(red) transcripts at early stage 5 at the rim of the germ disc (white dots). The lower panel shows the DNA fluorescence image. The inset contains an illustration of an embryo to show the orientation and the magnified region. (d) Expression ofAt-hh(purple) andAt-otd(red) transcripts at mid-stage 6 in the anterior marginal region of the nascent germ band. Left panels are the magnified view of the boxed region in the right panel, and the lower one shows the DNA fluorescence image. White dots show the anterior margin. (e) Detection of anAt-hhstripe in a tracked cell clone. An embryo having a cell clone labelled by FITC–dextran (green) more than two cells away from the rim of the germ disc (white dots) at early stage 5 (left panel) was fixed at early stage 7 and stained forAt-hhtranscripts (purple) and FITC–dextran (pink) (middle and right panels). The middle panel is a magnified view of the boxed region in the right panel. White dots show the anterior margin. Arrowheads indicate theAt-hhstripe (c–e). Scale bars, 100 μm ina, 50 μm inc–e. A, anterior; Ce, cephalic lobe; Ch, chelicera; Ex, extraembryonic tissue; L, leg; P, posterior; Pp, pedipalp. Figure 2: Movement of the At-hh expression stripe from the rim of the germ disc. ( a ) Tracking of a small cell clone labelled by microinjection of RITC–dextran (red). The live embryo was photographed at stages indicated. The rim of the germ disc near the clone is dotted (early stage 5). Arrows indicate the developing Ch and Pp segments. ( b ) Schematic diagram of Achaearanea development highlighting the transformation of the germ disc into a segmented germ band. The tracked cell clone shown in a is depicted in red. Approximate time after egg laying is shown. ( c ) Expression of At-hh (purple) and At-otd (red) transcripts at early stage 5 at the rim of the germ disc (white dots). The lower panel shows the DNA fluorescence image. The inset contains an illustration of an embryo to show the orientation and the magnified region. ( d ) Expression of At-hh (purple) and At-otd (red) transcripts at mid-stage 6 in the anterior marginal region of the nascent germ band. Left panels are the magnified view of the boxed region in the right panel, and the lower one shows the DNA fluorescence image. White dots show the anterior margin. ( e ) Detection of an At-hh stripe in a tracked cell clone. An embryo having a cell clone labelled by FITC–dextran (green) more than two cells away from the rim of the germ disc (white dots) at early stage 5 (left panel) was fixed at early stage 7 and stained for At-hh transcripts (purple) and FITC–dextran (pink) (middle and right panels). The middle panel is a magnified view of the boxed region in the right panel. White dots show the anterior margin. Arrowheads indicate the At-hh stripe ( c – e ). Scale bars, 100 μm in a , 50 μm in c – e . A, anterior; Ce, cephalic lobe; Ch, chelicera; Ex, extraembryonic tissue; L, leg; P, posterior; Pp, pedipalp. Full size image We examined the spatial relationships between the At-hh and At-otd expression patterns during early head development. The transcripts for At-hh and At-otd were co-expressed across 1–2 cells (in width) at the rim of the germ disc in early stage 5 ( Fig. 2c ). Despite cell internalization, At-hh - and At-otd -expression remained localized to the rim of the germ disc until the beginning of stage 6. Previous studies have found that as the germ disc begins to undergo morphological changes to form the germ band, the At-hh stripe shifts its relative position away from the anterior margin of the nascent germ band (the rim of the germ disc) towards the posterior (the centre of the germ disc) [23] , [27] . In the present study, double staining for At-hh and At-otd revealed that the shifting At-hh stripe was maintained at the posterior limit of the At-otd expression domain ( Fig. 2d ), which expands along the anteroposterior (AP) axis. Although this At-hh expression was considered dynamic in a previous study [23] , the authors did not exclude the possibility that the relative shifting of the At-hh stripe may result from cell movement or cell recruitment. To examine the dynamic properties of the At-hh -gene-expression stripe, we used a combination of cell clone tracking and molecular staining. A labelled cell clone that had been more than two cells away from the germ-disc rim at early stage 5 was intersected by an At-hh stripe detected in the presumptive head ectoderm at early stage 7 ( Fig. 2e ). This result, together with the expression data presented above, suggested that, from early stage 5 to early stage 7, more central (or posterior) cells progressively began to express At-hh , and cells located at more peripheral (or anterior) positions, presumably including future mesoderm cells, stopped expressing At-hh . Thus, we concluded that, at least during stage 6, the At-hh stripe travels some distance posteriorly as a wave. However, it was not easy to determine when and where the posterior movement of the At-hh stripe stops, despite a gene expression boundary being formed between the head and thoracic regions (see below). Repeated splitting of an At-hh gene expression stripe To follow the fate of the travelling At-hh stripe in the spider-head ectoderm, we took advantage of the simultaneous development of sibling embryos within an egg sac. Embryos were fixed at intervals of 2 h from the beginning of stage 7 (the time point defined as 0 h) over a period of 10 h (up to early stage 8) and were then double-stained for At-hh and At-otd or At-Deformed ( At-Dfd ) [27] ( Fig. 3 ). At-Dfd is a reliable marker of the thoracic region [30] , and its expression domain was complementary to the At-otd expression domain at early stage 7, but not at stage 8 ( Fig. 3a ). At the 0-h time point, the At-hh stripe exhibited the form of an arched line ∼ 2–4 cells wide that coincided with the posterior limit of the At-otd -expression domain, adjacent to the At-Dfd -expression domain ( Fig. 3b–d ). At the subsequent time points, the At-hh stripe overlapping with the At-otd expression domain broadened and nearly simultaneously or subsequently underwent insertion of an At-hh -negative domain, often exhibiting a pattern similar to an open mouth ( Fig. 3b–d , 2, 4 h). Various transient patterns were observed among embryos fixed at the 2-h and 4-h time points ( Supplementary Fig. S2 ), indicating that At-hh expression was disappearing from the middle regions of the stripe, a process that we refer to as 'splitting'. This splitting event was followed by shifting of the relative positions of the resulting stripes along the AP axis. Importantly, the anterior stripe remained At-otd positive, whereas the other stripe was At-otd negative. Only the At-otd -positive At-hh stripe underwent another cycle of splitting ( Fig. 3b , 6–10 h). These two cycles of splitting of gene expression stripes, each of which took roughly 4 h, accounted for the three At-hh stripes observed later in the head ectoderm ( Fig. 3b–d , 10 h), with the three stripes corresponding to the posterior portions of the Pp and Ch segments and the cephalic lobe (in this order starting from the posterior side). 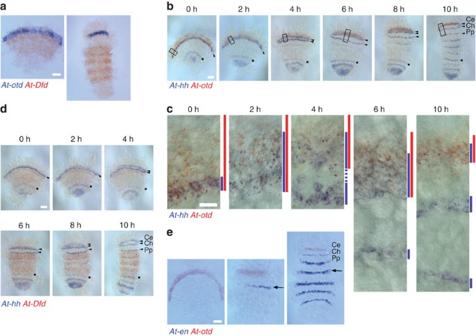Figure 3: Repeated splitting of theAt-hhstripe associated withAt-otdexpression. (a) Comparison of theAt-otd(purple) andAt-Dfd(red) expression domains in embryos at early stage 7 (left) and stage 8 (right). (b) Embryos from a single egg sac that were fixed at 2-h intervals and stained forAt-hh(purple) andAt-otd(red). The first fixation was performed at early stage 7 (0 h). Arrowheads indicateAt-hhstripes increasing in number in the presumptive head ectoderm. Dots indicate theAt-hhstripe corresponding to the L4 segment. (c) Differential interference contrast images of the five regions boxed inb. Blue and red lines on the right of each panel indicate the ranges of theAt-hhandAt-otdexpression domains, respectively. (d) Embryos from the same pools as inbstained forAt-hh(purple) andAt-Dfd(red) transcripts. TheAt-hhstripes are labelled in the same way as inb. (e) Embryos stained forAt-en(purple) andAt-otd(red) transcripts. Stage 6 (left), mid stage 7 (middle), and early stage 8 (right). Arrows indicate anAt-enstripe that is likely to correspond to the L1 segment. All embryos are oriented anterior towards the top. Ce, cephalic lobe; Ch, chelicera; Pp, pedipal. Scale bars, 100 μm ina,b,d,e; 20 μm inc. Figure 3: Repeated splitting of the At-hh stripe associated with At-otd expression. ( a ) Comparison of the At-otd (purple) and At-Dfd (red) expression domains in embryos at early stage 7 (left) and stage 8 (right). ( b ) Embryos from a single egg sac that were fixed at 2-h intervals and stained for At-hh (purple) and At-otd (red). The first fixation was performed at early stage 7 (0 h). Arrowheads indicate At-hh stripes increasing in number in the presumptive head ectoderm. Dots indicate the At-hh stripe corresponding to the L4 segment. ( c ) Differential interference contrast images of the five regions boxed in b . Blue and red lines on the right of each panel indicate the ranges of the At-hh and At-otd expression domains, respectively. ( d ) Embryos from the same pools as in b stained for At-hh (purple) and At-Dfd (red) transcripts. The At-hh stripes are labelled in the same way as in b . ( e ) Embryos stained for At-en (purple) and At-otd (red) transcripts. Stage 6 (left), mid stage 7 (middle), and early stage 8 (right). Arrows indicate an At-en stripe that is likely to correspond to the L1 segment. All embryos are oriented anterior towards the top. Ce, cephalic lobe; Ch, chelicera; Pp, pedipal. Scale bars, 100 μm in a , b , d , e ; 20 μm in c . Full size image Unlike in the head region, we observed no splitting pattern related to At-hh expression in the thoracic region. Three At-hh stripes of gene expression, corresponding to the L1-L3 segments, appeared nearly simultaneously from mid-stage 7 to early stage 8 ( Fig. 3b,d , 8, 10 h). An At-hh stripe corresponding to the L4 segment formed at the posterior end of the At-Dfd expression domain in stage 6 ( Fig. 3d , 0 h). The origins of the At-hh stripes for the opisthosomal segments seemed to be associated with the cycles of appearance and disappearance of At-hh expression at the centre of the caudal lobe ( Fig. 3b,d ). These observations imply that the mode of segmentation differs in the head, thoracic and opisthosomal regions. Furthermore, in contrast to At-hh , expression of another segment polarity gene homologue At-engrailed ( At-en ) [31] , was first detected at mid-to-late stage 7 ( Fig. 3e ). This At-en stripe seemed to correspond to the L1 segment. In the head and opisthosomal regions, the initiations of At-en expression were much later than those of At-hh expression, suggesting that At-en is not involved in the early steps of spider-head segmentation. Stripe splitting is accompanied by convergent extension To characterize the splitting process associated with the At-hh gene expression stripe in the head ectoderm at the cellular level, we monitored cell movements and cell divisions using live embryos locally expressing a fusion protein consisting of a nuclear localization signal (NLS) and tdEosFP (NLS-tdEosFP) ( n =4). Photoconversion of tdEosFP facilitated cell tracking. We analysed a representative dataset that covered 14.5 h of development starting from late stage 5 ( Fig. 4a,b ; Supplementary Movie 2 ). This analysis revealed that a period of ∼ 4.5 h (with few cell divisions) occurred between two 5-hr periods during which the cell number nearly doubled ( Fig. 4c ). During these three successive periods, the aspect ratio (length/width) of the labelled area progressively increased. Importantly, the cell counts across the width (the dorsoventral axis) of the labelled area decreased during the last two periods, indicating that oriented cell rearrangement in the epithelium contributed to elongating the AP axis of the head ectoderm, a typical convergent extension movement. 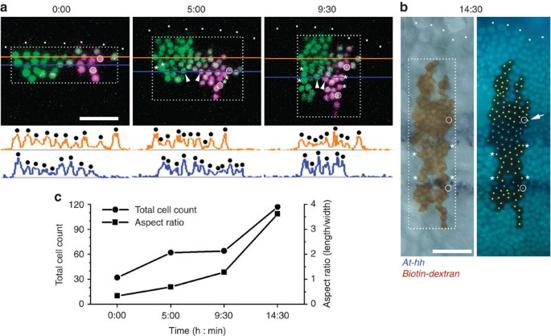Figure 4: Splitting of the headAt-hhstripe in epithelium undergoing convergent extension. (a) Time-lapse observation of a cell clone expressing NLS-tdEosFP in the presumptive head ectoderm. The tdEosFP was photoconverted from the green (shown in green) to the red state (shown in purple) in a part of the cell clone just before time-lapse observation was performed, which started at late stage 5. A series of 10 optical sections (7.76 μm thickness) was collected every 10 min, and shown are projections of the optical sections collected at the times indicated (h:min). Arrowheads indicate two cells that were undergoing rearrangement to become adjacent to each other. Fluorescence intensity profiles along the orange and blue lines are shown below the photos to assist cell counting. (b) Detection ofAt-hhstripes in the observed embryo that was placed in the fixative at∼14:30, which was 10 min after the last images were collected. The left panel shows expression ofAt-hhtranscripts (purple) and the cell lineage tracer biotin–dextran (brown), and the right shows the DNA fluorescence image.At-hh–positive and –negative cells in the labelled area are marked by light blue and yellow dots, respectively, although the signal was ambiguous in the cell indicated by the arrow. There were 22 labelled cells in theAt-hh-negative domain between the twoAt-hhstripes. Asterisks indicate the cells at the corners of theAt-hhnegative region between the twoAt-hhstripes (b) and their ancestral cells (a), and circles indicate the cells at the anterior and posterior ends of the two stripes (b) and their ancestral cells (a). White dots indicate the anterior margin of the nascent germ band. Scale bars, 50 μm. (c) Graph showing changes in the total cell count and aspect ratio (length/width) for the rectangles shown inaandbof the labelled area. Figure 4: Splitting of the head At-hh stripe in epithelium undergoing convergent extension. ( a ) Time-lapse observation of a cell clone expressing NLS-tdEosFP in the presumptive head ectoderm. The tdEosFP was photoconverted from the green (shown in green) to the red state (shown in purple) in a part of the cell clone just before time-lapse observation was performed, which started at late stage 5. A series of 10 optical sections (7.76 μm thickness) was collected every 10 min, and shown are projections of the optical sections collected at the times indicated (h:min). Arrowheads indicate two cells that were undergoing rearrangement to become adjacent to each other. Fluorescence intensity profiles along the orange and blue lines are shown below the photos to assist cell counting. ( b ) Detection of At-hh stripes in the observed embryo that was placed in the fixative at ∼ 14:30, which was 10 min after the last images were collected. The left panel shows expression of At-hh transcripts (purple) and the cell lineage tracer biotin–dextran (brown), and the right shows the DNA fluorescence image. At-hh –positive and –negative cells in the labelled area are marked by light blue and yellow dots, respectively, although the signal was ambiguous in the cell indicated by the arrow. There were 22 labelled cells in the At-hh -negative domain between the two At-hh stripes. Asterisks indicate the cells at the corners of the At-hh negative region between the two At-hh stripes ( b ) and their ancestral cells ( a ), and circles indicate the cells at the anterior and posterior ends of the two stripes ( b ) and their ancestral cells ( a ). White dots indicate the anterior margin of the nascent germ band. Scale bars, 50 μm. ( c ) Graph showing changes in the total cell count and aspect ratio (length/width) for the rectangles shown in a and b of the labelled area. Full size image Furthermore, in situ hybridization following the live observation revealed that the monitored cell clone was intersected by two separate At-hh stripes of gene expression ( Fig. 4b ). Cell tracing in the time-lapse movie suggested that the cells that covered the two At-hh stripes at the last time point (14.5 h) came from a line of approximately two cell widths at the 0-h time point (corresponding to late stage 5) and a line of approximately four cell widths at the 5-h time point (corresponding to late stage 6) ( Fig. 4a,b , circles) and, similarly, that the cells that comprised the At-hh -negative region between the At-hh gene expression stripes came from a line of approximately two cell widths at the 5-h time point ( Fig. 4a,b , asterisks). At late stage 6, before entering the first splitting cycle, the At-hh stripe was usually observed as a line ∼ 2–4 cell wide in essentially the same pattern as shown in Figure 3b–d , 0 h. These observations clearly show that the occurrence of an At-hh -negative domain between the two At-hh stripes during the splitting cycle is due to dynamic repression of At-hh expression accompanied by cell rearrangement in the surface epithelial layer, not by recruitment of At-hh -negative cells from other cell layers. We deduce from the time course of the development of the At-hh expression patterns ( Fig. 3 ) that the timing of the first splitting event of the At-hh gene expression stripe corresponds to the second proliferative period (between the 9.5-h and 14.5-h time points). However, because locally enhanced rates of cell division were not observed ( Fig. 4a,b ; Supplementary Movie 2 ), it is unlikely that the expansion of the emerging At-hh -negative domain results from regulation of cell division patterns. It is technically difficult to determine when each stripe of At-hh expression is settled in lineage-restricted cell populations. Role of At-otd for maintaining dynamic At-hh expression In general, the use of parental RNA interference (pRNAi) has limitations in cases where knockdown of a target gene in the entire embryo prevents development at earlier stages than the developmental event of interest occurs. In a previous study [23] , knockdown of At-otd by pRNAi was found to cause persistent localization of the At-hh stripe at the anterior margin of the nascent germ band. Here we observed that persistence of the At-hh stripe was concomitant with a failure in the normal specification of the At-Dfd -negative head region ( Supplementary Fig. S3 ). In the case of At-otd pRNAi, it was impossible to investigate the role of At-otd during the travelling and splitting of the At-hh stripe. To investigate the mechanisms underlying spider-head segmentation, we applied embryonic RNA interference (eRNAi) to Achaearanea embryos for the first time. Double-stranded RNAs (dsRNAs) for target genes, together with cell lineage tracers, were introduced into single blastomeres at the 32- to 128-cell stages. We confirmed that eRNAi produced cell-autonomous effects in Achaearanea with respect to the stability of target transcripts in the cytoplasm ( Supplementary Fig. S4 ). Two different dsRNAs were prepared for each gene and microinjected to confirm the production of gene-specific phenotypes ( Supplementary Table S1 ; Methods). The results obtained with only one of the two dsRNAs for each target gene are shown. In control eRNAi experiments, dsRNA for the jellyfish green fluorescent protein gene ( gfp ) was injected, which had no effects on the expression patterns of the target genes ( Fig. 5a ; Supplementary Fig. S5 ) or At-hh , regardless of the location of the cell clones into which the dsRNA was introduced ( Fig. 5b ; presumptive head ectoderm, n =12 (including cell clones covering the germ disc rim, n =7); thoracic and opisthosomal ectoderm, n =8). In At-otd eRNAi experiments, when the dsRNA was introduced in the thoracic and opisthosomal regions, the At-hh expression patterns were not affected ( Fig. 5c ; n =7). However, when the At-otd eRNAi cell clones covered the germ disc rim, similar, though local, defects compared with those caused by At-otd pRNAi were observed ( Fig. 5d ; 100%, n =7). This finding is consistent with the suggestion that At-otd is not essential for the initiation of At-hh expression but is required for the relative shifting of the At-hh stripe in the anterior terminal region [23] . This local prevention of the movement of the At-hh stripe resulted in parallel progression of head segmentation in two separate regions without affecting the development of thoracic At-hh stripes ( Fig. 5d ). More importantly, when the At-otd eRNAi cell clones were located in the presumptive head ectoderm (slightly removed from the germ disc rim), the At-hh stripe was allowed to begin travelling but was broken into two adjacent stripes by the clones ( Fig. 5e ; 100%, n =10). This unexpected phenotype was explained simply by loss of At-hh expression in the At-otd eRNAi cell clones. The separated At-hh stripes independently developed characteristic 'splitting' patterns with sizes adjusted to the smaller fields ( Fig. 5e ). Taken together, these results suggest that At-otd is required to maintain At-hh expression during the travelling and splitting phases and that the At-otd -positive At-hh stripe serves as a generative zone for the spider-head segments. 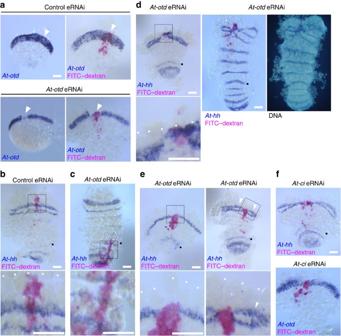Figure 5:At-otdactivity is required to maintain dynamicAt-hhexpression in the presumptive head ectoderm. (a) Detection ofAt-otdtranscripts in embryos microinjected with controlgfpdsRNA (upper panels) andAt-otdXEdsRNA (lower panels). Each embryo was photographed before (left) and after (right) staining for the lineage tracer FITC–dextran (pink). Arrowheads indicate areas where the lineage tracer and presumably the dsRNAs were introduced. (b) Control (gfp) eRNAi embryo stained forAt-hhtranscripts (purple) and the cell-lineage tracer FITC–dextran (pink), which was detected in the presumptive head ectoderm. Embryos shown in the following panels were stained in the same way as this embryo, unless otherwise indicated. (c)At-otdeRNAi embryo in which the labelled cell clone (pink) extended from the L4 segment to the caudal lobe. (d) TwoAt-otdeRNAi embryos that experienced having a labelled clone (pink) at the anterior margin of the nascent germ band at stages 6 and 7. The embryo in the left panel was fixed at stage 7, and that in the middle and right was allowed to develop until stage 8 and fixed for staining. The right panel shows the DNA fluorescence image. (e)At-otdeRNAi embryos in which the labelled clone (pink) was slightly removed from the anterior margin (white dots). The right embryo was slightly older than the left one. Arrowheads in the right panel indicate the adjacentAt-hhstripes that each exhibited a characteristic splitting pattern with sizes adjusted to the fields. (f)At-cieRNAi embryos; the lower one was stained forAt-otdtranscripts (purple) and the cell-lineage tracer FITC–dextran (pink). All embryos in this figure were at germ band-forming stages (corresponding to stage 7) except the embryo in right and middle panels ofd, which was at stage 8. Boxed areas in the upper panels are magnified in the lower panels (b,c,e, left column ofd). White dots indicate the anterior margin (b,d,e), and black dots indicate theAt-hhstripe at the L4 segment (b–f). Scale bars, 100 μm. Figure 5: At-otd activity is required to maintain dynamic At-hh expression in the presumptive head ectoderm. ( a ) Detection of At-otd transcripts in embryos microinjected with control gfp dsRNA (upper panels) and At-otdXE dsRNA (lower panels). Each embryo was photographed before (left) and after (right) staining for the lineage tracer FITC–dextran (pink). Arrowheads indicate areas where the lineage tracer and presumably the dsRNAs were introduced. ( b ) Control ( gfp ) eRNAi embryo stained for At-hh transcripts (purple) and the cell-lineage tracer FITC–dextran (pink), which was detected in the presumptive head ectoderm. Embryos shown in the following panels were stained in the same way as this embryo, unless otherwise indicated. ( c ) At-otd eRNAi embryo in which the labelled cell clone (pink) extended from the L4 segment to the caudal lobe. ( d ) Two At-otd eRNAi embryos that experienced having a labelled clone (pink) at the anterior margin of the nascent germ band at stages 6 and 7. The embryo in the left panel was fixed at stage 7, and that in the middle and right was allowed to develop until stage 8 and fixed for staining. The right panel shows the DNA fluorescence image. ( e ) At-otd eRNAi embryos in which the labelled clone (pink) was slightly removed from the anterior margin (white dots). The right embryo was slightly older than the left one. Arrowheads in the right panel indicate the adjacent At-hh stripes that each exhibited a characteristic splitting pattern with sizes adjusted to the fields. ( f ) At-ci eRNAi embryos; the lower one was stained for At-otd transcripts (purple) and the cell-lineage tracer FITC–dextran (pink). All embryos in this figure were at germ band-forming stages (corresponding to stage 7) except the embryo in right and middle panels of d , which was at stage 8. Boxed areas in the upper panels are magnified in the lower panels ( b , c , e , left column of d ). White dots indicate the anterior margin ( b , d , e ), and black dots indicate the At-hh stripe at the L4 segment ( b – f ). Scale bars, 100 μm. Full size image Moreover, phenotypes similar to those obtained from At-otd eRNAi were produced by performing eRNAi against At-cubitus interruptus ( At-ci ) ( Fig. 5f ; 100%, n =8 for clones covering the germ disc rim and n =7 for clones removed from the germ disc rim in the presumptive head region), a homologue of Drosophila ci ( Supplementary Fig. S6 ), which encodes a transcription factor that mediates the transduction of Hh signalling [32] . In At-ci eRNAi cell clones, At-otd expression was abrogated or greatly reduced ( Fig. 5f ; 100%, n =12). These results suggest that At-hh activity promotes At-otd expression via At-ci , while the At-otd activity promotes At-hh expression to maintain the head generative zone. Role of another Hh signalling target for promoting splitting To identify targets of Hh signalling other than At-otd , we carried out a microarray-based screen for genes that were downregulated in At-hh pRNAi embryos at late stage 5 ( Supplementary Table S2 ). A homologue of the Drosophila pair-rule gene odd-paired ( opa ) [33] , At-opa ( Supplementary Fig. S6 ), emerged as a putative target of Hh signalling in this screen. At-opa transcripts were detected in a broad marginal region of the germ disc covering the presumptive head ectoderm at late stage 5 ( Fig. 6a ); consistent with the microarray data, this expression was missing in At-hh pRNAi embryos ( Fig. 6a ). Later, relatively strong expression of At-opa transcripts was persistently observed at and near the At-otd -positive At-hh stripe, whereas weaker levels of stripe expression appeared in forming germ bands ( Fig. 6b ; Supplementary Fig. S7 ). pRNAi against At-opa caused a delay in axial elongation and simultaneously impaired the splitting of the head At-hh stripe without disrupting the travelling process or the anterior terminal patterning ( Fig. 6c ; Supplementary Fig. S3 ). This situation resembles what is seen during Drosophila pair-rule patterning, which is coupled with convergent extension [34] . A similar delay in axial elongation was also observed in At-otd pRNAi embryos ( Supplementary Fig. S3 ). 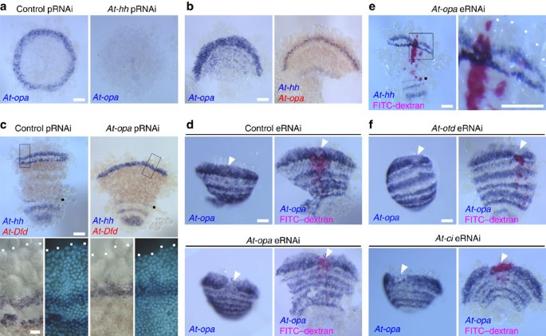Figure 6:At-opaactivity is required to promote stripe splitting and its expression is regulated by segmentation genes. (a) Control (gfp) (left) andAt-hh(right) pRNAi embryos at late stage 5 stained forAt-opatranscripts. (b) Embryos at early stage 7 single-stained forAt-opatranscripts (left) and double-stained forAt-hh(purple) andAt-opa(red) transcripts (right). (c) Control (gfp) (left) andAt-opa(right) pRNAi embryos at germ band-forming stages stained forAt-hh(purple) andAt-Dfd(red) transcripts. The boxed areas in the upper panels are magnified in the lower panels; the right ones are fluorescence images of DNA staining. The right embryo is∼6 holder than the left embryo (seeMethods). Note that the number ofAt-hhstripes for the L4 (black dots) and more posterior segments is an alternative indicator of developmental stage. (d) Detection ofAt-opatranscripts in embryos microinjected with controlgfpdsRNA (upper panels) andAt-opaFdsRNA (lower panels). Each embryo was photographed before (left) and after (right) staining for the lineage tracer FITC–dextran (pink). Arrowheads indicate areas where the lineage tracer and, presumably, the dsRNAs were introduced. (e)At-opaeRNAi embryo stained forAt-hhtranscripts (purple) and the cell lineage tracer FITC–dextran (pink). The boxed area in the left panel is magnified in the right panel. (f) Detection ofAt-opatranscripts inAt-otdeRNAi (upper panels) andAt-cieRNAi (lower panels) embryos. Staining and photographing were performed in the same way as ind. White dots indicate the anterior margin of the germ band, and black dots indicate theAt-hhstripe in the L4 segment (c,e). Embryos shown ind–fwere at early or mid stage 7. Scale bars, 20 μm in the lower panel ofc, 100 μm in other panels. Figure 6: At-opa activity is required to promote stripe splitting and its expression is regulated by segmentation genes. ( a ) Control ( gfp ) (left) and At-hh (right) pRNAi embryos at late stage 5 stained for At-opa transcripts. ( b ) Embryos at early stage 7 single-stained for At-opa transcripts (left) and double-stained for At-hh (purple) and At-opa (red) transcripts (right). ( c ) Control ( gfp ) (left) and At-opa (right) pRNAi embryos at germ band-forming stages stained for At-hh (purple) and At-Dfd (red) transcripts. The boxed areas in the upper panels are magnified in the lower panels; the right ones are fluorescence images of DNA staining. The right embryo is ∼ 6 holder than the left embryo (see Methods ). Note that the number of At-hh stripes for the L4 (black dots) and more posterior segments is an alternative indicator of developmental stage. ( d ) Detection of At-opa transcripts in embryos microinjected with control gfp dsRNA (upper panels) and At-opaF dsRNA (lower panels). Each embryo was photographed before (left) and after (right) staining for the lineage tracer FITC–dextran (pink). Arrowheads indicate areas where the lineage tracer and, presumably, the dsRNAs were introduced. ( e ) At-opa eRNAi embryo stained for At-hh transcripts (purple) and the cell lineage tracer FITC–dextran (pink). The boxed area in the left panel is magnified in the right panel. ( f ) Detection of At-opa transcripts in At-otd eRNAi (upper panels) and At-ci eRNAi (lower panels) embryos. Staining and photographing were performed in the same way as in d . White dots indicate the anterior margin of the germ band, and black dots indicate the At-hh stripe in the L4 segment ( c , e ). Embryos shown in d – f were at early or mid stage 7. Scale bars, 20 μm in the lower panel of c , 100 μm in other panels. Full size image To more directly investigate the role of At-opa in head segmentation, we used eRNAi ( Fig. 6d ). In At-opa eRNAi cell clones located in the presumptive head ectoderm, the At-hh stripe was prevented from splitting ( Fig. 6e ; 90%, n =10). These results suggest that At-opa activity promotes stripe splitting in the head generative zone. Regulation of At-opa striped pattern formation To investigate the role of At-otd in the regulation of At-opa expression, we examined At-otd eRNAi cell clones. In cell clones located in the thoracic and opisthosomal region, At-opa expression was not affected ( n =8). In contrast, in cell clones located in the presumptive head ectoderm, the levels of At-opa expression were considerably reduced, and the head At-opa stripes failed to separate ( Fig. 6f ; 90%, n =10), suggesting that At-otd activity is required in the presumptive head ectoderm for normal development of the striped pattern of At-opa expression. Similar phenotypes were observed in At-ci eRNAi cell clones located in the presumptive head ectoderm ( Fig. 6f ; 100%, n =11). Furthermore, depletion of At-opa transcripts by At-opa pRNAi resulted in a uniform pattern of At-opa transcription ( Supplementary Fig. S8 ). This suggests that the activity of At-opa is required for its striped pattern of transcription to be established. We have identified the splitting of gene expression stripes as a mode of segmentation in A. tepidariorum that occurs in the presumptive head ectoderm using microinjection-based techniques, such as cell labelling and eRNAi. This segmentation type presents several unique features compared with Drosophila blastoderm subdivision and vertebrate oscillatory segmentation (Compare Fig. 7 with Fig. 1a,b ). First, movement of a gene expression wave is a critical step in specifying the segmentation field. This was suggested by the observation that stripe-travelling defects caused by At-otd pRNAi (ref. 23 ; Supplementary Fig. S3 ) and eRNAi ( Fig. 5d ) were followed by failures in the formation of the head region. Second, there is a narrow (stripe-shaped) generative zone from which new repetitive units form in a specific sequence. Segmentation in this zone would resemble those in the presomitic mesoderm of vertebrate embryos and the posterior growth zone of short-germ arthropod embryos in that they show temporal repetition. Third, development of segmental gene expression patterns is associated with convergent extension elongating the tissue axis. Fourth, the changing patterns of gene expression involved in segmentation mimic the travelling and peak splitting of waves that have been observed in numerical simulations of a class of autocatalytic reaction–diffusion systems in a growing field ( Fig. 1d ). 'Stripe splitting', a behaviour similar to self-replication ( Fig. 1d ), is distinguished from the oscillatory generation of new waves in the terminal region ( Fig. 1b ) and from the insertion of new waves at a distance from pre-existing waves ( Fig. 1c ). On the basis of these observed features, we suggest that spider-head segmentation is of particular importance in understanding the relationships among the diverse modes of animal segmentation, and we categorize it as the split-type segmentation. 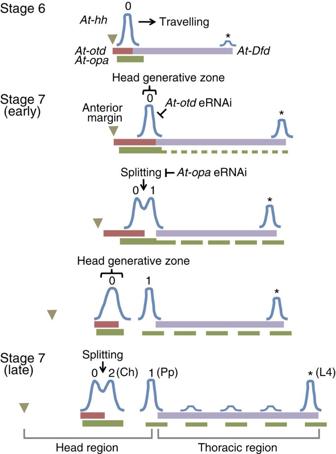Figure 7: Schematic illustrations showing the changes in gene expressions involved inAchaearaneahead segmentation. The expression domains ofAt-hh(blue waves),At-otd(brown boxes),At-opa(green boxes), andAt-Dfd(purple boxes) along the AP axis at five successive stages of development are illustrated. Only the head and thoracic regions are shown. TheAt-otd-positive wave ofAt-hhexpression, marked by '0', is defined as the generative zone for the Pp and Ch segments, which form by stripe splitting in that order and are indicated by '1' and '2', respectively. The anterior margin of the forming germ band (closed triangles) and theAt-hhexpression stripe related to the L4 segment (asterisks) are also indicated.At-otdeRNAi inhibitsAt-hhexpression in the head generative zone, andAt-opaeRNAi prevents theAt-otd-positiveAt-hhstripe from splitting. In earlier stages (late stage 5 and early stage 6),At-otdeRNAi inhibits the departure of theAt-hhstripe from the rim of the germ disc, but this fact is not shown. Figure 7: Schematic illustrations showing the changes in gene expressions involved in Achaearanea head segmentation. The expression domains of At-hh (blue waves), At-otd (brown boxes), At-opa (green boxes), and At-Dfd (purple boxes) along the AP axis at five successive stages of development are illustrated. Only the head and thoracic regions are shown. The At-otd -positive wave of At-hh expression, marked by '0', is defined as the generative zone for the Pp and Ch segments, which form by stripe splitting in that order and are indicated by '1' and '2', respectively. The anterior margin of the forming germ band (closed triangles) and the At-hh expression stripe related to the L4 segment (asterisks) are also indicated. At-otd eRNAi inhibits At-hh expression in the head generative zone, and At-opa eRNAi prevents the At-otd -positive At-hh stripe from splitting. In earlier stages (late stage 5 and early stage 6), At-otd eRNAi inhibits the departure of the At-hh stripe from the rim of the germ disc, but this fact is not shown. Full size image Here we have characterized some of the molecular mechanisms associated with spider-head segmentation. Taken together with the results of our previous study [27] , these findings suggest that Hh signalling has central roles in AP axis formation and subsequent head segmentation. We found that although expression of At-otd and At-opa is controlled by Hh signalling via At-ci , their activities are required to dynamically regulate the distribution patterns of Hh-signalling sources. These findings led us to propose that spider-head segmentation requires an autoregulatory signalling network in which At-hh , At-ci , At-otd and At-opa participate ( Fig. 8 ). It is important to note that the posterior limit of the At-otd expression domain continues to be closely associated with the anterior-most At-hh stripe ( Figs 3b,c and 7 ), suggesting that At-otd transcription is activated by short-range activity of Hh signalling. In contrast, at least at late stage 5 and late stage 6 ( Figs 6a,b and 7 ), the posterior limit of the broad At-opa -expression domain is away from the At-hh -signalling source, suggesting that At-opa transcription is activated by longer range signals. Positive feedback regulation of Hh signalling by At-otd seems to contribute to maintaining the spider-head generative zone, whereas At-opa , encoding a Zic family transcription factor, may be a key gene required to generate stripe-splitting dynamics in the head generative zone. 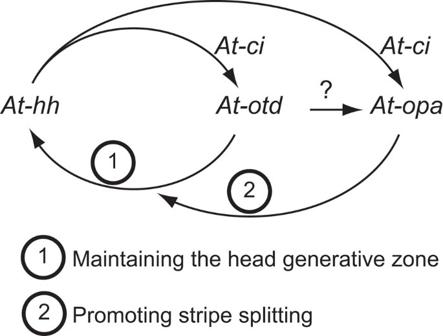Figure 8: A model for mechanisms underlying spider-head segmentation. An autoregulatory signalling network in whichAt-hh,At-ci,At-otd, andAt-opaparticipate is proposed. Expression ofAt-otdandAt-opais controlled by short- and longer range activities ofAt-hh, respectively, viaAt-ci, and activities ofAt-otdandAt-opaare required for the dynamic regulation ofAt-hhexpression during head segmentation.At-otdactivity mediates positive feedback to maintain the head generative zone, andAt-opaactivity promotes theAt-hh—At-otdcircuit to enter the splitting phase through an as yet unknown mechanism in the head generative zone. The stripe splitting may involve coordinated regulation of gene expression and cell rearrangement.At-otdmay directly and/or indirectly regulate levels ofAt-opaexpression and the development of its pattern. Figure 8: A model for mechanisms underlying spider-head segmentation. An autoregulatory signalling network in which At-hh , At-ci , At-otd , and At-opa participate is proposed. Expression of At-otd and At-opa is controlled by short- and longer range activities of At-hh , respectively, via At-ci , and activities of At-otd and At-opa are required for the dynamic regulation of At-hh expression during head segmentation. At-otd activity mediates positive feedback to maintain the head generative zone, and At-opa activity promotes the At-hh — At-otd circuit to enter the splitting phase through an as yet unknown mechanism in the head generative zone. The stripe splitting may involve coordinated regulation of gene expression and cell rearrangement. At-otd may directly and/or indirectly regulate levels of At-opa expression and the development of its pattern. Full size image Peak splitting of gene expression waves has been characteristically observed in numerical simulations of activator-depleted substrate systems, which assume local self-enhancement (autocatalysis) and depletion of a substance required for the self-enhancement [6] , [35] . The At-hh — At-otd reciprocal positive regulation might mimic local self-enhancement, whereas At-opa may act as a cofactor involved in the self-enhancement. If the At-Opa protein is consumed, depletion of this product might promote the At-hh — At-otd circuit to enter the splitting phase. With respect to this possibility, mammalian Zic proteins may act synergistically with Gli proteins, which are Ci homologues, to enhance the transduction of Hh signalling [36] . Zic and Gli family proteins share a highly conserved zinc finger domain ( Supplementary Fig. S6 ) and have cooperative roles in multiple developmental processes [37] , [38] . Alternatively, the At-Opa product might have a substantial inhibitory effect on Hh signalling preferentially at sites where its signalling activities are saturated. Zic family proteins also act antagonistically with Gli family proteins [36] . These hypotheses need to be tested. An important aspect of our findings is that the observed splitting of gene expression stripes may require coordinated regulation of gene expression and cell rearrangement. Knockdown of At-otd and At-opa appeared to delay convergent extension. At-otd and At-opa activities may mediate interactions of multiple signalling pathways that coordinate pattern formation and cell movements. The types of signalling pathways, other than Hh signalling, involved in this gene expression stripe splitting are a key issue to be studied in the future. Identification of shared genetic components suggests an evolutionary link between spider stripe-splitting segmentation and Drosophila Bicoid-based segmentation. The proposed autoregulatory signalling network for the stripe-splitting segmentation contrasts with the hierarchical cascades of maternal, gap and pair-rule genes associated with Drosophila blsastoderm subdivision while sharing Hh-signalling components with the segment polarity network. The activities of the Drosophila pair-rule genes prepattern the segments and activate the segment polarity gene network [17] , in which the Hh and Wingless signalling pathways have reciprocal regulatory interactions to determine correct cell fates within each segment [39] , [40] . Importantly, roles of these signalling pathways are restricted to the terminal steps in Drosophila segmentation. Curiously, the gene expression stripe splitting is somewhat similar to pair-rule patterning that has been observed in some short-germ arthropod embryos, where domains of gene expression are progressively resolved into segmental stripes [23] , [24] . Our findings and these facts may provide hints about the evolution of mechanisms of pair-rule patterning. Mutations affecting network structures of segmentation genes could have led to diversification of strategies for arthropod segmentation [4] . As mentioned above, the spider embryo exhibits at least three distinct modes of segmentation depending on the body part. Intriguingly, Drosophila subdivision is achieved by distinct mechanisms in the head and trunk regions [3] , [41] , [42] . Increases in the number of stripes or patches of segment polarity gene homologue expression have been observed in the developing head region of Drosophila and other arthropod embryos [43] , [44] , [45] , [46] , [47] , where split-like patterning events may occur. Furthermore, the spider-head generative zone is analogous to the vertebrate midbrain–hindbrain boundary zone, which is considered the head organizer, in which both zones are defined by the posterior limits of the expression domains of the otd / otx homologues [48] . Animal segmentation will continue to be a challenging subject in studying how developmental strategies diversified during animal body plan evolution. Spiders This work was performed according to institutional animal care and use committee guidelines. Laboratory stocks of the house spider A. tepidariorum were maintained at 25 °C. The development of sibling embryos was monitored to evaluate the quality of the embryos used in our experiments. Developmental stages were described previously [25] , [28] , [29] . Embryo staining Embryos from a single egg sac were fixed at 2-h intervals from the beginning of stage 7 and pooled as a series of 0 h to 10 h samples. Embryos shown in Figures 3b–d and 6b , and Supplementary Figures S2 and S7 were derived from this series. Embryo fixation and whole-mount in situ hybridization were performed, as described previously [28] , [31] . Fluorescein isothiocyanate (FITC)–dextran in fixed samples was visualized using an alkaline phosphatase-conjugated sheep anti-FITC antibody (1:1000, dilution; Roche) and the Vector Red substrate (Vector). Biotin–dextran was visualized using the VECTASTAIN Elite standard ABC kit (Vector). Most samples were counterstained with 4′,6-diamidino-2-phenylindole (DAPI; Sigma-Aldrich). Embryos were examined using an SZX12 fluorescence stereomicroscope (Olympus) equipped with a colour charge-coupled device camera (C7780-10; Hamamatsu Photonics) and/or an Axiophot2 fluorescence microscope equipped with differential interference contrast optics (Carl Zeiss). Microinjection Embryos at appropriate stages were dechorionated with commercial bleach, placed on glass slides, covered with halocarbon oil 700 (Sigma), and subjected to microinjection as described [25] . A 1 μg μl −1 solution of FITC–dextran (MW 500,000, Sigma-Aldrich) or rhodamine B isothiocyanate (RITC)–dextran (MW 70,000, Sigma-Aldrich) was injected into 32- to 128-cell stage embryos. Live embryos were photographed using the fluorescence stereomicroscope. Plasmid construction and mRNA preparation The pSP64 poly(A) vector (Promega) was modified to replace the Eco RI site after the poly A sequence with a Not I site. This plasmid was designated pSP64-polyA-NotI+. A blunt-ended Xho I- Bam HI fragment of the pcDNA3-Flag1-td-EosFP plasmid (Molecular Biotechnology) was inserted into the Sma I site of pSP64-polyA-NotI+ to produce pSP64-tdEosFP-polyA-NotI+. A Hind III (blunt-ended)- BamHI fragment encoding the NLS (the amino acid sequence, MAKIPPKKKRKVED) was inserted between the Hinc II and Bam HI sites of pSP64-tdEosFP-polyA-NotI+. The resulting plasmid was designated pSP64-NLS-tdEosFP-polyA-NotI+ and was cut with Not I for use as a template for in vitro transcription. Capped sense messenger RNA was synthesized using the mMESSAGE mMACHINE SP6 Kit (Ambion) according to the manufacturer's instructions. Time-lapse observations Embryos at the 32-cell stage were injected with a mixture of NLS-tdEosFP mRNA (0.25 μgμl −1 ). and biotin–dextran (MW 70,000, Sigma-Aldrich, 1.0 μg μl −1 ). For photoconversion of tdEosFP, small areas of the embryos were ultraviolet irradiated for less than 3 min under the Axiophot2 fluorescence microscope using a band-pass excitation filter (Chroma No. 31022, BP 395±20) and a X40 objective. Neither the expression of NLS-tdEosFP nor the ultraviolet irradiation resulted in any detectable toxic effect on development. Time-lapse microscopy was performed using the TCS SPE confocal system (Leica). Images were processed using Leica LAS-AF ver. 2.21, ImageJ ver. 1.44 (NIH) and Adobe Photoshop CS2 software. Microarray-based screen of spider genes We obtained 22,812 expressed sequence tags (ESTs) sequenced from the 5′ end from five complementary DNA (cDNA) libraries of A. tepidariorum embryos. These sequences were deposited in the DNA Data Bank of Japan under accession numbers FY216297–FY225483 and FY368221–FY381845. To design microarray probes, 13,655 non-redundant sequences were selected from the EST data. Using these sequences and a few extra sequences, 40 mer oligonucleotide probes were designed using OligoArray 2.1 software [49] and embedded in CombiMatrix custom microarrays (12K×2). Total RNA was extracted from two different populations of late-stage 5 embryos derived from different egg sacs produced by a single female 1 day before (normal) and 20 days after ( At-hh pRNAi) the first injection of At-hh1 dsRNA. This female was given a total of four injections of ∼ 1.5 μl of At-hh1 dsRNA solution (2 μg μl −1 ) at 2–3 day intervals. cRNA labelled with Cy3 (normal) or Cy5 ( At-hh pRNAi) was prepared from 2 μg of total RNA using the RNA Transcript SureLABEL Core Kit (TaKaRa). cRNA probes were hybridized to microarrays in hybridization buffer (5× saline-sodium citrate buffer, 0.1% sodium dodecyl sulphate, 10% formamide) at 42 °C for 16–20 h. Microarray slides were scanned using a GenePix 4000B Scanner (Molecular Devices), and the obtained images were analysed using Array-Pro Analyzer version 4.5 (Media Cybernetics). The quantitative data were subjected to loess normalization. To validate this microarray experiment, probes for At-hh and At-otd served as positive controls; probes for an α-catenin homologue, an elongation factor 1α homologue, and an H3 histone homologue were used as negative controls ( Supplementary Table S2 ). The intensity ratio values in the spots for two EST clones representing sequences homologous to Drosophila opa , eS6_d1_54_H12 (FY376203) and eS7_SB_031_C08 (FY380182) were as low as those for the positive controls. These EST clones were clustered with another EST clone At_eW_022_A24 (FY223306). The microarray dataset was deposited in the Gene Expression Omnibus database under accession number GSE26468. cDNA and genomic DNA cloning The EST clone At_eW_022_A24 and an extra cDNA clone obtained by 5′ rapid amplification of cDNA ends (RACE) were used to determine the sequence of the entire coding region of At-opa . A short sequence homologous to Drosophila ci was originally found in an EST clone eS6_d1_31_A04 (FY374226). A full-length cDNA clone for At-ci was obtained by 5′ and 3′ RACE and cDNA library screening. Analyses with BLASTP and Mega version 4.0 (ref. 50 ) confirmed that the predicted proteins encoded by At-opa and At-ci were zinc finger proteins that belong to the Opa/Zic and Ci/Gli subfamilies, respectively ( Supplementary Fig. S6 ). cDNA clones covering the entire coding region of an A. tepidariorum homologue of six3 , designated At-six3-1 , were obtained by PCR using degenerate primers and 5′ and 3′ RACE. The sequences are available from the DNA database of Japan under the accession numbers At-opa , AB605264; At-ci , AB605263; and At-six3-1 , AB605265. A genomic DNA clone sharing a sequence with the At-opa cDNA clone was obtained by screening an A. tepidariorum genomic library (λdash II) constructed during this study. This clone covered at least a part of an intron following an exon/intron boundary that is evolutionarily conserved at the junction of the zinc finger 3 and 4 coding regions [51] . A 1-kb fragment within this intron was used to prepare an intron probe to detect At-opa pre-mRNA. RNAi DNA templates for dsRNA synthesis were prepared by PCR with primers bearing the T7 or Sp6 promoter sequence. dsRNA was synthesized using a MEGAscript kit (Ambion) as described [52] . gfp dsRNA was used as a control. To validate the specificity of the RNAi effects, we prepared two different dsRNAs per gene, which were derived from non-overlapping regions of the cDNA or regions with a minimum overlap (four nucleotides). For At-otd and At-opa RNAi, longer dsRNAs were also prepared and tested to confirm the consistency of the results. Information on the dsRNAs used in this study is summarized in Supplementary Table S1 . Reduced expression levels of the target transcripts were confirmed by in situ hybridization and/or quantitative reverse transcription polymerase chain reaction ( Supplementary Table S1 ). pRNAi was performed by injecting dsRNA into the opisthosoma of females using a pulled glass capillary, as described in ref. 31 . Individual females were given multiple injections of 1.5–2.0 μl of a dsRNA solution (2 μg μl −1 ) at 2- to 3-day intervals ( At-opa1 , At-opaF , At-otd1 , At-otdXE , At-hh1 and At-hh2 dsRNAs, four or five injections; At-opaH and gfp dsRNAs, seven injections). At-opa pRNAi and At-otd pRNAi reduced the speed of the transition from the germ disc to the germ band. To exclude the possibility that the defects described for these pRNAi embryos resulted from developmental delays, we examined these embryos at slightly later stages than the control embryos. The embryos shown in Figure 6c (right) and Supplementary Figure S3a,d,f were ∼ 6 h older than the control embryos shown in Figure 6c (left) and Supplementary Figure S3e,g . In the eRNAi experiments, a mixture of dsRNA (0.3–0.4 μg μl −1 ) and FITC–dextran (0.4–0.8 μg μl −1 ) or a mixture of dsRNA (0.4 μg μl −1 ) and RITC-dextran (0.8 μg μl −1 ) plus biotin–dextran (MW 10,000, Sigma-Aldrich, 0.4 μg μl −1 ) (for the experiment shown in Supplementary Fig. S4 ) was microinjected into 32- to 128-cell stage embryos. At the time of injection, the fates of the injected cells were not predictable because of the spherical symmetry of the early Achaearanea embryo. At late stage 5, morphologically normal embryos in which labelled cell clones were located at target sites of the germ disc epithelium were selected under the fluorescence microscope for analysis. As it was not possible to strictly control the injection volume, the amount of dsRNA incorporated into embryonic cells (as indicated by the fluorescence intensity of incorporated FITC–dextran) slightly varied from embryo to embryo. However, such variations had little effect on the experimental results. In the pRNAi and/or eRNAi experiments for each gene, the same results were independently obtained with the two dsRNAs. The results shown here were obtained with one of the dsRNAs for each gene: At-opaF , At-otdXE , At-ci1 , and At-hh1 (against At-opa , At-otd , At-ci , and At-hh , respectively). In the eRNAi experiments, we obtained the same results in 80% or more of embryos examined ( n ≥5) with the other dsRNA for each gene. Accession codes: The A. tepidariorum EST data have been deposited in the DNA Data Bank of Japan under accession numbers FY216297 to FY225483 and FY368221 to FY381845 . The microarray data have been deposited in the Gene Expression Omnibus database under accession number GSE26468. Nucleotide sequences for the A. tepidariorum genes are available from the DNA Data Bank of Japan under the following accession numbers: At-opa , AB605264 ; At-ci , AB605263 ; At-six3-1 , AB605265 . How to cite this article: Kanayama, M. et al . Travelling and splitting of a wave of hedgehog expression involved in spider-head segmentation. Nat. Commun. 2:500 doi: 10.1038/ncomms1510 (2011).